Control of response reliability by parvalbumin-expressing interneurons in visual cortex The responses of visual cortical neurons to natural stimuli are both reliable and sparse. These properties require inhibition, yet the contribution of specific types of inhibitory neurons is not well understood. Here we demonstrate that optogenetic suppression of parvalbumin (PV)- but not somatostatin (SOM)-expressing interneurons reduces response reliability in the primary visual cortex of anaesthetized and awake mice. PV suppression leads to increases in the low firing rates and decreases in the high firing rates of cortical neurons, resulting in an overall reduction of the signal-to-noise ratio (SNR). In contrast, SOM suppression generally increases the overall firing rate for most neurons, without affecting the SNR. Further analysis reveals that PV, but not SOM, suppression impairs neural discrimination of natural stimuli. Together, these results reveal a critical role for PV interneurons in the formation of reliable visual cortical representations of natural stimuli. Inhibition plays an essential role in cortical processing of sensory information [1] , [2] , [3] . Previous pharmacological studies have demonstrated that GABAergic inhibition is critical for both gain control and stimulus selectivity of cortical neurons [2] , [4] , [5] , [6] . Moreover, response reliability [7] , [8] is also regulated by inhibitory circuits. For example, in the primary visual cortex (V1), co-stimulation of the classical- and non-classical receptive field (RF) of pyramidal neurons causes an increase in response reliability and sparseness; these effects were associated with increased inhibitory inputs [9] . In the middle temporal visual area, blocking GABAergic inhibition reduces response reliability and direction selectivity of cortical neurons [10] . In the auditory cortex, balanced but delayed inhibition produces precise spike timing of tone-evoked cell responses [11] . In the hippocampus, feed-forward inhibition can enforce the temporal fidelity of pyramidal cell spiking [12] . Similar inhibitory circuits were also found to increase the temporal precision of neuronal response in the somatosensory cortex [13] . These studies all suggest that neural response reliability is tightly controlled by inhibitory networks. Although GABAergic interneurons account for ∼ 20% of cortical neurons [14] , [15] , they are diverse in terms of morphological, synaptic, molecular and electrophysiological properties [14] , [16] , [17] . Studying how each type of inhibitory neuron contributes to cortical processing is essential to understanding brain function under physiological and pathological conditions [1] , [2] . Based on the expression of calcium-binding proteins and neuropeptides, interneurons can be classified into distinct groups [14] , [16] , [18] , [19] , among which parvalbumin (PV)- and somatostatin (SOM)-expressing neurons constitute a large fraction [14] , [19] . Recent studies have used optogenetic techniques to examine how the activities of PV and SOM interneurons influence properties such as cortical response gain, stimulus selectivity and spatial integration [20] , [21] , [22] , [23] , [24] , [25] . However, the effect of specific type of inhibitory interneuron on cortical response reliability remains uncharacterized. PV interneurons, which are the most prevalent type of interneuron in the cortex [14] , [16] , are implicated in neurological disorders such as autism and epilepsy [26] , [27] , [28] . Sensory-evoked responses are unreliable and signal-to-noise ratios (SNRs) are weak in sensory cortices in autism [29] . It is therefore important to directly examine the contribution of PV interneurons to cortical response reliability and SNR during sensory processing. In the present study, we use multi-electrode recording in mouse V1 to measure cortical neural responses to repeated presentations of movies with natural scenes, with and without optogenetic suppression of PV or SOM interneurons. In both anaesthetized and awake mice, we find that only PV suppression results in reduced response reliability and SNR of V1 neurons. In particular, PV suppression results in an increase in the firing rate to stimuli that evoke small responses and a decrease in the firing rate to stimuli that evoke large responses. On the other hand, SOM suppression is accompanied by an increase in response rate across all stimuli. Finally, we show that PV suppression functionally results in impaired neural discriminability of different natural stimuli. Together, our results demonstrate that PV interneurons critically contribute to the response reliability and visual coding of cortical neurons. To optically suppress the activity of PV or SOM interneurons, we conditionally expressed the light-sensitive proton pump Archeorhodopsin (Arch) [30] , [31] in PV or SOM neurons in mouse V1 by injecting adeno-associated virus into PV-Cre [32] or SOM-Cre [33] mice. Immunostaining showed that Arch-GFP was expressed across almost all cortical layers, with the expression of Arch restricted to PV- or SOM-positive neurons ( Fig. 1 ). To measure the effects of Arch suppression, we used multichannel silicon probe to record V1 activity near the virus injection site. Based on their spike waveforms, neurons were grouped into broad-spiking and narrow-spiking cells ( Supplementary Fig. 1 ), corresponding to putative excitatory and putative inhibitory neurons [34] . As strong suppression of PV interneurons can cause epileptiform activity [21] , [35] , we chose a moderate level of PV suppression to avoid aberrant activity in the cortex ( Supplementary Fig. 2 ). 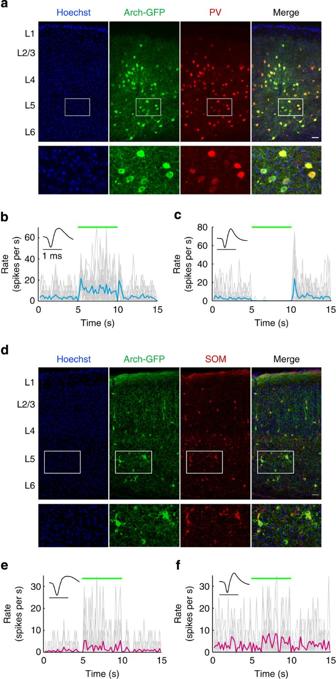Figure 1: Effects of optogenetically suppressing PV- and SOM-expressing neurons. (a) Fluorescent images of cells immunopositive for PV and Arch-GFP. Top, coronal section of V1 from aPV-Cremouse injected with Cre-dependent Arch-GFP adeno-associated virus (AAV)–vector. Blue, nuclear staining with Hoechst; green, Arch-GFP-expressing cells (anti-GFP immunostaining); red, PV-expressing cells (anti-PV immunostaining). Scale bar, 40 μm. Bottom, magnification of the boxed region at top. Note that Arch-GFP was strongly expressed in both granular and infragranular layers, and Arch expression only occurred in PV-expressing cells. (b) Spontaneous spiking response of a putative excitatory neuron (broad-spiking, spike waveform shown in the inset) with and without PV suppression. Grey traces, responses in different trials; blue trace, response averaged over all trials. Green bar indicates the duration of laser stimulation. (c) Spontaneous spiking response of a putative PV neuron with and without PV suppression, same as described inb. (d) Fluorescent images of cells immunopositive for SOM (red) and Arch-GFP (green). Top, coronal section of V1 from aSOM-Cremouse injected with Cre-dependent Arch-GFP AAV–vector. Bottom, magnification of the boxed region at top. Similar as described ina. Scale bar, 40 μm. (e) Effect of SOM suppression on the spontaneous response of a putative excitatory cell, similar as described inb. Magenta trace, response averaged over all trials. (f) Effect of SOM suppression on the spontaneous response of a narrow-spiking cell, similar as described inb. Figure 1: Effects of optogenetically suppressing PV- and SOM-expressing neurons. ( a ) Fluorescent images of cells immunopositive for PV and Arch-GFP. Top, coronal section of V1 from a PV-Cre mouse injected with Cre-dependent Arch-GFP adeno-associated virus (AAV)–vector. Blue, nuclear staining with Hoechst; green, Arch-GFP-expressing cells (anti-GFP immunostaining); red, PV-expressing cells (anti-PV immunostaining). Scale bar, 40 μm. Bottom, magnification of the boxed region at top. Note that Arch-GFP was strongly expressed in both granular and infragranular layers, and Arch expression only occurred in PV-expressing cells. ( b ) Spontaneous spiking response of a putative excitatory neuron (broad-spiking, spike waveform shown in the inset) with and without PV suppression. Grey traces, responses in different trials; blue trace, response averaged over all trials. Green bar indicates the duration of laser stimulation. ( c ) Spontaneous spiking response of a putative PV neuron with and without PV suppression, same as described in b . ( d ) Fluorescent images of cells immunopositive for SOM (red) and Arch-GFP (green). Top, coronal section of V1 from a SOM-Cre mouse injected with Cre-dependent Arch-GFP AAV–vector. Bottom, magnification of the boxed region at top. Similar as described in a . Scale bar, 40 μm. ( e ) Effect of SOM suppression on the spontaneous response of a putative excitatory cell, similar as described in b . Magenta trace, response averaged over all trials. ( f ) Effect of SOM suppression on the spontaneous response of a narrow-spiking cell, similar as described in b . Full size image PV but not SOM suppression reduces response reliability We characterized the effect of photo suppression on the responses of putative excitatory (broad spiking) cells to visual stimulation. We presented time-varying natural scene movies, while optogenetically suppressing PV or SOM cells during interleaved trials. We first examined responses in anaesthetized mice. As shown by the spike trains of an example putative excitatory cell obtained during control (that is, no optogenetic stimulation) trials in Fig. 2a , natural movies evoked sparse episodes of spiking that exhibited similar temporal patterns over trials. PV suppression increased this neuron’s spiking response to the movie ( Fig. 2a , right). For the population of putative excitatory cells studied, PV suppression caused a significant increase in visual stimulus-evoked firing rate ( P =1.2 × 10 −9 , n =98 broad-spiking cells, Wilcoxon signed-rank test; Fig. 2b ). To quantify the reliability for each cell during control trials or during optogenetic stimulation, we computed the Pearson correlation coefficient (CC) of its responses (binned at the stimulus frame rate) between each pair of trials and averaged the CCs over all pair-wise combinations of trials [36] . We found that PV suppression significantly reduced the response reliability of putative excitatory neurons ( P =7.9 × 10 −9 , Wilcoxon signed-rank test; Fig. 2c ). As anaesthesia can affect the activity of inhibitory neurons [20] , we also examined the effect of optogenetic stimulation in awake, head-fixed mice ( Fig. 2d , a putative excitatory cell). Similar to the results obtained in anaesthetized mice, PV suppression in awake mice resulted in a significant increase in firing rate ( P =0.01, n =28 broad-spiking cells, Wilcoxon signed-rank test; Fig. 2e ) and a significant decrease in the CC of responses ( P =7.4 × 10 −5 , Wilcoxon signed-rank test; Fig. 2f ). The decrease in CC resulting from PV suppression was consistently observed for responses analysed using different bin sizes ranging from 20 to 300 ms ( Supplementary Fig. 3 ). As a control, optogenetic stimulation itself affected neither the firing rate nor the response reliability of V1 neurons in animals that did not receive viral injection ( Supplementary Fig. 4 ). Thus, PV interneurons play a critical role in controlling the response reliability of cortical neurons. 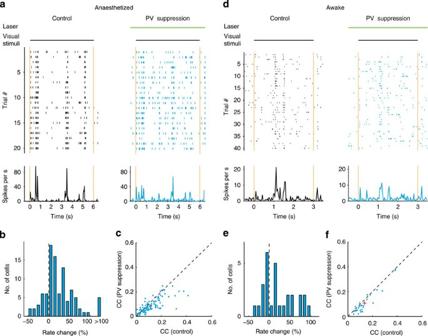Figure 2: PV suppression decreases response reliability. (a) Responses of a putative excitatory cell in an anaesthetized mouse to repeated stimulation of a 6-s movie (raster and PSTH). Left, without optogenetic stimulation, CC=0.41; right, with optogenetic PV suppression, CC=0.17. For this cell, ΔCC=−0.24, change of evoked firing rate=7.3% and Δspontaneous firing rate=1.3 spikes per second. Optogenetic stimulation started 0.5 s before the onset of natural movie and terminated 0.5 s after the offset of movie. Horizontal black bar, duration of natural movie. Horizontal green bar, duration of optogenetic stimulation. Yellow vertical lines indicate the onset and offset of movie. (b) Histogram of firing-rate changes for putative excitatory cells induced by PV suppression in anaesthetized mice. (c) Summary of response reliability measured by between-trial CC with and without PV suppression in anaesthetized mice (n=98 putative excitatory cells,P=7.9 × 10−9, Wilcoxon signed-rank test). (d) Responses of a putative excitatory cell in an awake mouse to repeated stimulation of a 3-s movie (raster and PSTH), similar to those described ina. Left, without optogenetic stimulation, CC=0.11; right, with optogenetic PV suppression, CC=0.06. For this cell, ΔCC=−0.05, change of evoked firing rate=0% and Δspontaneous firing rate=0.3 spike per second. (e) Histogram of firing rate changes for putative excitatory cells induced by PV suppression in awake mice. (f) Summary of response reliability with and without PV suppression in awake mice (n=28 putative excitatory cells,P=7.4 × 10−5, Wilcoxon signed-rank test). CCs were computed using the responses binned at the stimulus frame rate. Error bars (plus symbols in panelscandf) represent±s.e.m. Figure 2: PV suppression decreases response reliability. ( a ) Responses of a putative excitatory cell in an anaesthetized mouse to repeated stimulation of a 6-s movie (raster and PSTH). Left, without optogenetic stimulation, CC=0.41; right, with optogenetic PV suppression, CC=0.17. For this cell, ΔCC=−0.24, change of evoked firing rate=7.3% and Δspontaneous firing rate=1.3 spikes per second. Optogenetic stimulation started 0.5 s before the onset of natural movie and terminated 0.5 s after the offset of movie. Horizontal black bar, duration of natural movie. Horizontal green bar, duration of optogenetic stimulation. Yellow vertical lines indicate the onset and offset of movie. ( b ) Histogram of firing-rate changes for putative excitatory cells induced by PV suppression in anaesthetized mice. ( c ) Summary of response reliability measured by between-trial CC with and without PV suppression in anaesthetized mice ( n =98 putative excitatory cells, P =7.9 × 10 −9 , Wilcoxon signed-rank test). ( d ) Responses of a putative excitatory cell in an awake mouse to repeated stimulation of a 3-s movie (raster and PSTH), similar to those described in a . Left, without optogenetic stimulation, CC=0.11; right, with optogenetic PV suppression, CC=0.06. For this cell, ΔCC=−0.05, change of evoked firing rate=0% and Δspontaneous firing rate=0.3 spike per second. ( e ) Histogram of firing rate changes for putative excitatory cells induced by PV suppression in awake mice. ( f ) Summary of response reliability with and without PV suppression in awake mice ( n =28 putative excitatory cells, P =7.4 × 10 −5 , Wilcoxon signed-rank test). CCs were computed using the responses binned at the stimulus frame rate. Error bars (plus symbols in panels c and f ) represent±s.e.m. Full size image In both anaesthetized and awake mice, photo suppression of SOM cells increased the visual stimulus-evoked responses of putative excitatory neurons ( P =1.7 × 10 −9 and 0.002, n =51 and 25 for anaesthetized and awake mice, respectively, Wilcoxon signed-rank test; Fig. 3a,b,d,e ). The distributions of change in firing rate of broad-spiking cells resulting from PV and SOM suppression were not significantly different ( Supplementary Fig. 5a ). However, SOM suppression did not have a significant effect on the CC of responses in either anaesthetized or awake mice ( P =0.66 and 0.51, Wilcoxon signed-rank test; Fig. 3c,f ). 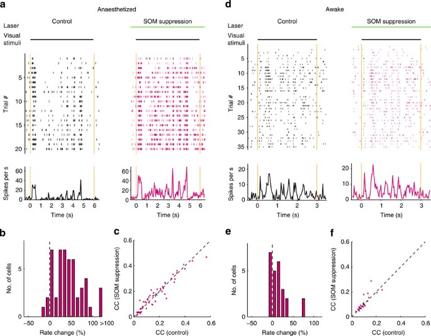Figure 3: SOM suppression does not alter response reliability. (a) Responses of a putative excitatory cell in an anaesthetized mouse to repeated stimulation of a 6-s movie (raster and PSTH). Left, without optogenetic stimulation; right, with optogenetic suppression of SOM interneurons. Same as described inFig. 2a. (b) Histogram of firing rate changes for putative excitatory cells induced by SOM suppression in anaesthetized mice. (c) Summary of response reliability with and without SOM suppression in anaesthetized mice (n=51 putative excitatory cells,P=0.66, Wilcoxon signed-rank test). (d) Responses of a putative excitatory cell in an awake mouse to repeated stimulation of a 3-s movie (raster and PSTH), similar to those described ina. (e) Histogram of firing rate changes for putative excitatory cells induced by SOM suppression in awake mice. (f) Summary of response reliability with and without SOM suppression in awake mice (n=25 putative excitatory cells,P=0.51, Wilcoxon signed-rank test). CCs were computed using the responses binned at the stimulus frame rate. Error bars (plus symbols in panelscandf) represent±s.e.m. Figure 3: SOM suppression does not alter response reliability. ( a ) Responses of a putative excitatory cell in an anaesthetized mouse to repeated stimulation of a 6-s movie (raster and PSTH). Left, without optogenetic stimulation; right, with optogenetic suppression of SOM interneurons. Same as described in Fig. 2a . ( b ) Histogram of firing rate changes for putative excitatory cells induced by SOM suppression in anaesthetized mice. ( c ) Summary of response reliability with and without SOM suppression in anaesthetized mice ( n =51 putative excitatory cells, P =0.66, Wilcoxon signed-rank test). ( d ) Responses of a putative excitatory cell in an awake mouse to repeated stimulation of a 3-s movie (raster and PSTH), similar to those described in a . ( e ) Histogram of firing rate changes for putative excitatory cells induced by SOM suppression in awake mice. ( f ) Summary of response reliability with and without SOM suppression in awake mice ( n =25 putative excitatory cells, P =0.51, Wilcoxon signed-rank test). CCs were computed using the responses binned at the stimulus frame rate. Error bars (plus symbols in panels c and f ) represent±s.e.m. Full size image The distributions of CC change (ΔCC, the CC measured with optogenetic stimulation minus that without optogenetic stimulation) were significantly different for PV and SOM suppression experiments ( P =1.1 × 10 −7 , Kolmogorov–Smirnov test; Supplementary Fig. 6 ). Analysis of covariance further revealed that the effects of PV and SOM suppression on response reliability were significantly different ( P =2.8 × 10 −6 , Supplementary Fig. 6 ). To control for the possibility that the different effects of PV and SOM suppression were due to sampling different neuron populations, we compared response properties on control trials with no optogenetic stimulation between the two populations. Neither firing rate nor response reliability was significantly different between the two populations ( Supplementary Fig. 5b,c ). Thus, the different effects of PV and SOM suppression could not be attributed to sampling from different underlying putative excitatory neuron populations. CC tends to increase with increasing firing rate [37] ; to control for this possible confound, we performed a spike rate equalization analysis [36] . For each trial, the firing rates with and without optogenetic stimulation were equalized by randomly adding spikes for the spike train with lower firing rate. Even after spike rate equalization, the decrease in CC was observed only for PV suppression but not for SOM suppression ( Supplementary Fig. 7 ). Thus, the decrease in CC during PV suppression could not be explained only by the increase in firing rate. To examine the laminar distribution of the effects, we performed current source density (CSD) analysis of the local field potential (LFP) responses evoked by flash stimuli to identify the location of cortical layer 4 ( Supplementary Fig. 8a ). We found that the decrease in CC induced by PV suppression was observed across all cortical layers ( P =2.2 × 10 −4 , 4.5 × 10 −5 and 9.8 × 10 −4 , n =26, 35 and 25 for supragranular, granular and infragranular layer, respectively, Wilcoxon signed-rank test), whereas the CCs for neurons in all layers remained unchanged by SOM suppression ( P =0.83, 0.9 and 0.45, n =17, 11 and 45 for supragranular, granular and infragranular layer, respectively, Wilcoxon signed-rank test; Supplementary Fig. 8b,c ). PV and SOM suppression differently affect high firing rates It has been shown that an increase in response reliability is associated with a selective increase in spiking during episodes of high firing probability [37] . Examination of the peristimulus time histograms (PSTHs) in Fig. 4a,b shows that PV suppression tended to result in a reduction in peak firing rates as opposed to an increase. To examine how the change in firing rate following interneuron suppression depends on baseline (that is, control) response level, we performed a robust linear regression between the responses with and without optogenetic suppression ( Fig. 4c,d ). For PV suppression, the slope of the linear fit was significantly smaller than one ( P =2.4 × 10 −10 and 0.002, n =98 and 28 for anaesthetized and awake mice, respectively, Wilcoxon signed-rank test) and the y intercept was significantly larger than zero ( P =3.0 × 10 −16 and 6.5 × 10 −6 for anaesthetized and awake mice, respectively, Wilcoxon signed-rank test; Fig. 4e ). We further separated the time bins in the PSTH into events and non-events using a threshold of 25% of the maximum response [37] , [38] . We found that PV suppression significantly decreased firing rates during events but increased the firing rates of non-events ( Supplementary Fig. 9a ). For SOM suppression, on the other hand, the slope of the linear fit between the responses with and without photo stimulation was not significantly different from one ( P =0.63 and 0.08, n =51 and 25 for anaesthetized and awake mice, respectively, Wilcoxon signed-rank test) and the y intercept was significantly larger than zero ( P =1.1 × 10 −9 and 3.2 × 10 −5 for anaesthetized and awake mice, respectively, Wilcoxon signed-rank test; Fig. 4e ). Thus, PV and SOM suppression have different effects on the visual stimulus-evoked firing rates: PV suppression tended to result in decreases in peak firing rates and increases in minimum firing rates, whereas SOM suppression tended to increase firing rates across all baseline levels. 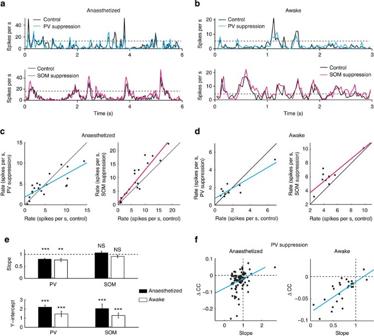Figure 4: PV and SOM suppression have different effects on peak firing rates. (a) Example PSTHs from anaesthetized mice. Upper, PSTH of a putative excitatory cell with (blue) and without (black) PV suppression. Lower, PSTH of a putative excitatory cell with (magenta) and without (black) SOM suppression. Dashed line: 25% of the maximum response measured without optogenetic stimulation. (b) Example PSTHs from awake mice. Same as described ina. (c) Relationship between the responses (binned at 300 ms) with and without optogenetic stimulation for two putative excitatory cells in anaesthetized mice. Left, with and without PV suppression. Right, with and without SOM suppression. Blue or magenta line, robust linear fit of the data; black line, the diagonal line. (d) Relationship between the responses (binned at 300 ms) with and without optogenetic stimulation for two putative excitatory cells in awake mice. Same as described inc. (e) Slope andyintercept for the robust linear fit between the responses with and without photo suppression. PV suppression:n=98 and 28 for anaesthetized and awake mice; SOM suppression:n=51 and 25 for anaesthetized and awake mice. (f) ΔCC versus slope for PV suppression (r=0.34,P=5.3 × 10−4for anaesthetized mice;r=0.79,P=4.7 × 10−7for awake mice). ΔCC: CC with PV suppression minus that without PV suppression. Error bars represent±s.e.m. ***P<0.0001, **P<0.01, Wilcoxon signed-rank test. Figure 4: PV and SOM suppression have different effects on peak firing rates. ( a ) Example PSTHs from anaesthetized mice. Upper, PSTH of a putative excitatory cell with (blue) and without (black) PV suppression. Lower, PSTH of a putative excitatory cell with (magenta) and without (black) SOM suppression. Dashed line: 25% of the maximum response measured without optogenetic stimulation. ( b ) Example PSTHs from awake mice. Same as described in a . ( c ) Relationship between the responses (binned at 300 ms) with and without optogenetic stimulation for two putative excitatory cells in anaesthetized mice. Left, with and without PV suppression. Right, with and without SOM suppression. Blue or magenta line, robust linear fit of the data; black line, the diagonal line. ( d ) Relationship between the responses (binned at 300 ms) with and without optogenetic stimulation for two putative excitatory cells in awake mice. Same as described in c . ( e ) Slope and y intercept for the robust linear fit between the responses with and without photo suppression. PV suppression: n =98 and 28 for anaesthetized and awake mice; SOM suppression: n =51 and 25 for anaesthetized and awake mice. ( f ) ΔCC versus slope for PV suppression ( r =0.34, P =5.3 × 10 −4 for anaesthetized mice; r =0.79, P =4.7 × 10 −7 for awake mice). ΔCC: CC with PV suppression minus that without PV suppression. Error bars represent±s.e.m. *** P <0.0001, ** P <0.01, Wilcoxon signed-rank test. Full size image We next examined whether the reduction in response reliability resulting from PV suppression is related to the changes in firing rate. Across the population, ΔCC was significantly correlated with the change in event firing rate ( r =0.6 and 0.75, P =5.9 × 10 −11 and 5.2 × 10 −6 for anaesthetized and awake mice, respectively; Supplementary Fig. 9b ), as well as with the slope of the regression between responses with and without optogenetic suppression ( r =0.34 and 0.79, P =5.3 × 10 −4 and 4.7 × 10 −7 for anaesthetized and awake mice, respectively; Fig. 4f ); ΔCC was not significantly correlated with the change in non-event firing rate ( r =0.02 and 0.1, P =0.84 and 0.63 for anaesthetized and awake mice, respectively; Supplementary Fig. 9c ). These results indicate that the reduction in response reliability during PV suppression may be largely attributable to the decreases in the responses of high firing rates. We further examined the effect of optogenetic suppression on the SNR of the responses. During movie stimulation, the event responses were likely to be evoked by stimuli that matched the RF properties of the neurons and thus could be considered as the signals. SNR was defined as the ratio between the mean firing rate of events and the s.d. of event firing rates over trials [29] . In both anaesthetized and awake mice, PV suppression significantly reduced the SNR of putative excitatory neurons ( P =7.0 × 10 −12 and 0.038 for anaesthetized and awake mice, respectively, Wilcoxon signed-rank test; Fig. 5a ). The PV suppression-induced change in SNR (ΔSNR, defined as the SNR measured with optogenetic suppression minus that without suppression) significantly correlated with the decrease in event firing rate ( r =0.87 and 0.88, P =1.3 × 10 −30 and 7.5 × 10 −10 for anaesthetized and awake mice, respectively; Supplementary Fig. 9d ). In contrast, SOM suppression did not significantly change SNR in either anaesthetized or awake mice ( P =0.85 and 0.48, respectively, Wilcoxon signed-rank test; Fig. 5b ). The distributions of ΔSNR were significantly different between PV and SOM suppression experiments ( P =9.8 × 10 −9 , Kolmogorov–Smirnov test; Supplementary Fig. 10 ). 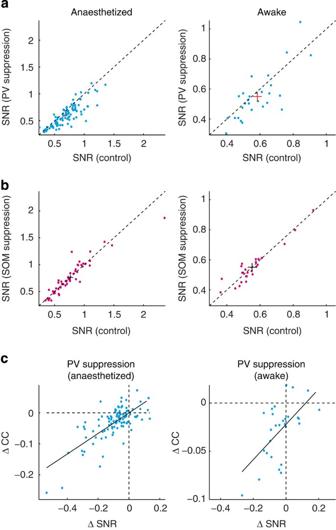Figure 5: PV but not SOM suppression decreases SNR in anaesthetized and awake mice. (a) Summary of SNR with and without PV suppression (P=7 × 10−12,n=98 for anaesthetized mice;P=0.038,n=28 for awake mice; Wilcoxon signed-rank test). (b) Summary of SNR with and without SOM suppression (P=0.85,n=51 for anaesthetized mice;P=0.48,n=25 for awake mice; Wilcoxon signed-rank test). (c) ΔCC versus ΔSNR for PV suppression (r=0.73,P=1.1 × 10−17for anaesthetized mice;r=0.61,P=6.2 × 10−4for awake mice). Error bars (plus symbols in panelsaandb) represent±s.e.m. Figure 5: PV but not SOM suppression decreases SNR in anaesthetized and awake mice. ( a ) Summary of SNR with and without PV suppression ( P =7 × 10 −12 , n =98 for anaesthetized mice; P =0.038, n =28 for awake mice; Wilcoxon signed-rank test). ( b ) Summary of SNR with and without SOM suppression ( P =0.85, n =51 for anaesthetized mice; P =0.48, n =25 for awake mice; Wilcoxon signed-rank test). ( c ) ΔCC versus ΔSNR for PV suppression ( r =0.73, P =1.1 × 10 −17 for anaesthetized mice; r =0.61, P =6.2 × 10 −4 for awake mice). Error bars (plus symbols in panels a and b ) represent±s.e.m. Full size image For PV suppression, ΔSNR was significantly correlated with ΔCC in both anaesthetized and awake mice ( r =0.73 and 0.61, P =1.1 × 10 −17 and 6.2 × 10 −4 , respectively; Fig. 5c,d ). Thus, the decrease in response reliability may be related to the reduction in SNR during PV suppression. We also quantified the response variability of event responses by computing the Fano factor (FF), which is the time average of the ratio between spike count variance and mean spike count. We found that PV suppression resulted in a significant increase in FF ( P =0.001, Wilcoxon signed-rank test; Supplementary Fig. 11a ), suggesting that PV interneuron suppression increased the trial-to-trial variability of event responses. In contrast, SOM suppression did not significantly change the response FF ( P =0.76, Wilcoxon signed-rank test; Supplementary Fig. 11b ). For PV suppression, we further determined the relationships among changes in CC, event response and SNR by computing Pearson partial CCs. We found that the reduction in CC was significantly correlated with the decrease in event response ( r =0.32, P =1.7 × 10 −4 , n =126 from both anaesthetized and awake mice) and the decrease in event response was significantly correlated with the decrease in SNR ( r =0.69, P =1.3 × 10 −19 , n =126). The correlation between decrease in CC and decrease in SNR was weak but significant ( r =0.17, P =0.03, n =126). Taken together, these results indicated that the decrease in response reliability and SNR during PV suppression could be attributed to the decrease in high-rate neuronal response. Both PV and SOM suppression reduce response sparseness We next examined the impact of PV or SOM suppression on neural selectivity for individual natural movies. To quantify the degree of selectivity, we used the measure of sparseness [9] , [39] , which approaches one for highly selective neurons and is near 0 for non-selective neurons. Both PV and SOM suppression significantly decreased the response sparseness ( P =1.6 × 10 −15 and n =126 for PV suppression and P =6.3 × 10 −8 and n =76 for SOM suppression, Wilcoxon signed-rank test; Fig. 6a,b ). The decrease in sparseness induced by PV suppression (−0.07±0.01, s.e.m.) was significantly larger than that induced by SOM suppression (−0.04±0.01, s.e.m., P =0.006, Wilcoxon rank-sum test). For both PV and SOM suppression, there was a significant negative correlation between the changes in sparseness and firing rate ( r =−0.5, P =3.3 × 10 −9 for PV suppression and r =−0.6, P =2.7 × 10 −8 for SOM suppression; Fig. 6c,d ), and a significant positive correlation between the changes in sparseness and CC ( r =0.31, P =3.5 × 10 −4 for PV suppression and r =0.35, P =0.002 for SOM suppression; Fig. 6e,f ). Partial correlation analysis showed that the change in sparseness was significantly correlated with both the change in firing rate ( r =−0.56, P =1.8 × 10 −11 for PV suppression and r =−0.57, P =1.2 × 10 −7 for SOM suppression) and the change in CC ( r =0.41, P =1.5 × 10 −6 for PV suppression and r =0.3, P =0.009 for SOM suppression).Thus, both PV and SOM interneurons contribute to sparseness of cortical neuron responses to natural movies. 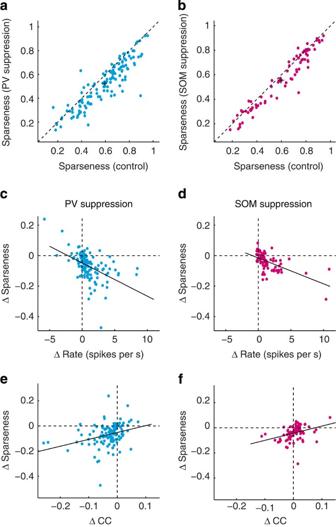Figure 6: Both PV and SOM suppression decrease sparseness in responses to natural stimuli. (a) Summary of response sparseness with and without PV suppression (P=1.6 × 10−15,n=126 from both anaesthetized and awake mice, Wilcoxon signed-rank test). (b) Summary of response sparseness with and without SOM suppression (P=6.3 × 10−8,n=76 from both anaesthetized and awake mice,Wilcoxon signed-rank test). (c) Change in sparseness induced by PV suppression significantly correlated with change in firing rate (r=−0.5,P=3.3 × 10−9). (d) Change in sparseness induced by SOM suppression significantly correlated with change in firing rate (r=−0.6,P=2.7 × 10−8). (e) Change in sparseness versus ΔCC for PV suppression (r=0.31,P=3.5 × 10−4). (f) Change in sparseness versus ΔCC for SOM suppression (r=0.35,P=0.002). Solid line, linear fit of the data. Error bars (plus symbols in panelsaandb) represent±s.e.m. Figure 6: Both PV and SOM suppression decrease sparseness in responses to natural stimuli. ( a ) Summary of response sparseness with and without PV suppression ( P =1.6 × 10 −15 , n =126 from both anaesthetized and awake mice, Wilcoxon signed-rank test). ( b ) Summary of response sparseness with and without SOM suppression ( P =6.3 × 10 −8 , n =76 from both anaesthetized and awake mice,Wilcoxon signed-rank test). ( c ) Change in sparseness induced by PV suppression significantly correlated with change in firing rate ( r =−0.5, P =3.3 × 10 −9 ). ( d ) Change in sparseness induced by SOM suppression significantly correlated with change in firing rate ( r =−0.6, P =2.7 × 10 −8 ). ( e ) Change in sparseness versus ΔCC for PV suppression ( r =0.31, P =3.5 × 10 −4 ). ( f ) Change in sparseness versus ΔCC for SOM suppression ( r =0.35, P =0.002). Solid line, linear fit of the data. Error bars (plus symbols in panels a and b ) represent±s.e.m. Full size image PV suppression impairs neural discrimination How does PV or SOM suppression affect the ability of V1 neurons to discriminate different stimuli? To address this issue, we quantified neural discrimination on the basis of single-trial responses using classification analysis [40] , [41] . We divided the movie into multiple segments and computed a response template for each segment by taking the average response across trials (see Methods). By estimating the similarity between a single-trial response in a movie segment and each response template on the basis of Euclidean distance, we assigned the single-trial response to one of the movie segments ( Fig. 7a ). Discrimination performance was defined as the percentage of trials that were correctly classified. We found that PV suppression significantly reduced neural discrimination performance ( P =4.0 × 10 −4 , n =126, Wilcoxon signed-rank test), and that the effect was significantly correlated with the reduction in response reliability ( r =0.3, P =7.0 × 10 −4 ; Fig. 7b ). In contrast, SOM suppression did not affect neural discrimination performance ( P =0.37, n =76, Wilcoxon signed-rank test; Fig. 7c ). Thus, PV interneurons play an important role in sculpting distinct cortical representations for different natural scenes. 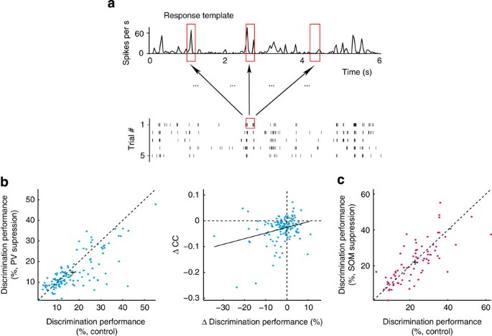Figure 7: PV suppression reduces neural discrimination between different natural stimuli. (a) Schematic illustration of the neural discrimination analysis. The single-trial response to a given stimulus segment (200 ms, red box) was classified as being generated by one of the segments on the basis of its Euclidean distances from the response templates of all segments (red boxes in the PSTH). The response template was defined by the response averaged across trials, excluding the trial used for discrimination. (b) Left, PV suppression reduced the discrimination performance (P=4.0 × 10−4,n=126, combining both anaesthetized and awake mice, Wilcoxon signed-rank test). Right, ΔCC versus change in discrimination performance for PV suppression (r=0.3,P=7.0 × 10−4). Solid line, linear fit of the data. (c) SOM suppression did not significantly impact discrimination performance (P=0.37,n=76, combining both anaesthetized and awake mice, Wilcoxon signed-rank test). Error bars (plus symbols in panelsbandc) represent±s.e.m. Figure 7: PV suppression reduces neural discrimination between different natural stimuli. ( a ) Schematic illustration of the neural discrimination analysis. The single-trial response to a given stimulus segment (200 ms, red box) was classified as being generated by one of the segments on the basis of its Euclidean distances from the response templates of all segments (red boxes in the PSTH). The response template was defined by the response averaged across trials, excluding the trial used for discrimination. ( b ) Left, PV suppression reduced the discrimination performance ( P =4.0 × 10 −4 , n =126, combining both anaesthetized and awake mice, Wilcoxon signed-rank test). Right, ΔCC versus change in discrimination performance for PV suppression ( r =0.3, P =7.0 × 10 −4 ). Solid line, linear fit of the data. ( c ) SOM suppression did not significantly impact discrimination performance ( P =0.37, n =76, combining both anaesthetized and awake mice, Wilcoxon signed-rank test). Error bars (plus symbols in panels b and c ) represent±s.e.m. Full size image In the present study, we found distinct effects of PV and SOM suppression on cortical representations of natural stimuli. PV suppression tended to result in an increase in low-rate neuronal responses and a reduction in high-rate neuronal responses, which were associated with a reduction in response reliability, SNR and response sparseness. SOM suppression tended to increase firing rates across all firing rate levels, which was associated with a reduction in response sparseness without significant changes in response reliability and SNR. Reliability of neuronal responses is important for the fidelity of sensory coding [7] . Previous studies have shown that cortical response reliability depends on visual experience [37] , the context of visual stimulation [9] and the brain state of the animal [36] , [42] , [43] . In the cat visual cortex, wide-field natural stimulation increases the reliability of pyramidal neurons and the effects are accompanied by an increase in inhibitory inputs, probably caused by the increased activity of fast-spiking (FS) interneurons [9] . Using an optogenetic approach, our study in the mouse visual cortex provides direct evidence that PV interneurons, which are typically FS [14] , [16] , contribute to the response reliability of putative excitatory pyramidal neurons. We found that the reduction in reliability during PV suppression was associated with a reduction in event firing rates and a decrease in SNR. A recent study in the hippocampus showed that increases in the activity of FS interneurons caused a reduction in feed-forward inhibition, leading to enhancement of SNR and fidelity of spike transmission in pyramidal neurons [44] . This decrease in feed-forward inhibition depended on the increase in FS spiking and potentially arised from synaptic depression of the FS-pyramidal synapse [44] . In the visual cortex, PV interneurons provide powerful inhibitory inputs to pyramidal neurons and PV-pyramidal synapses may also exhibit frequency-dependent synaptic depression [45] , [46] . In our study, natural stimuli resulted in temporally sparse neural responses that contained distinct episodes of high firing rates. Optogenetic stimulation of Arch in PV-expressing interneurons significantly reduced the firing rates of narrow-spiking cells ( Supplementary Fig. 1g ). Further analysis of the narrow-spiking cells showed that their event responses could be decreased by >10 Hz during photo stimulation ( Supplementary Fig. 12 ). The decrease in spiking of PV interneurons during high firing rate episodes may be associated with less synaptic depression of PV-pyramidal synapses, resulting in enhanced feed-forward inhibition. Our finding that PV suppression reduced the event firing rates for putative pyramidal neurons is in accordance with the speculation that PV suppression increased feed-forward inhibition during events. During visual stimulation that evokes low rates, PV-pyramidal synapses may exhibit negligible depression. In such cases, PV suppression may decrease the inhibitory inputs to pyramidal neurons, leading to disinhibition and enhancement of low-rate neuronal responses. Two recent studies examined the impact of PV or SOM activation on stimulus selectivity to grating stimuli. Although one study showed that PV but not SOM activation enhanced stimulus selectivity [22] , another reported that SOM activation sharpened but PV activation preserved selectivity [23] . Although this difference may be due to differences in the protocols of optogenetic activation as well as basic differences in the visual stimuli themselves [22] , [23] , [47] , [48] , our present results demonstrated that both PV and SOM interneurons contribute to response sparseness during natural stimulation. Although we found that PV suppression reduced the natural visual stimulus-evoked maximum firing rates and increased minimum firing rates, a recent study using drifting gratings showed that PV suppression increased pyramidal responses regardless of baseline level [21] . Natural stimuli usually evoke sparser and stronger transient responses than grating stimuli [37] , [39] , [49] . Higher firing rates can lead to stronger depression of PV-pyramidal synapses, which might contribute to the different effects of PV suppression on pyramidal responses. Another difference between the studies is that here we used extended period of optogenetic stimulation. The period when both optogenetic stimulation and visual stimulation occurred was 6 or 3 s in our study and 1–2 s in the previous study [21] . A third difference is in the laminar location of the virus injection. The virus was injected at a depth of 300–500 μm in the previous study [21] , with the expression of Arch restricted to layer 2/3. In our study, the viral injection site was at 500–750 μm below the cortical surface and Arch was expressed across all cortical layers, with strong expression in both granular and infragranular layers ( Fig. 1 ). As the same type of GABAergic interneurons in different cortical layers can exhibit different output connectivity and electrophysiological properties [50] , the function of inhibitory neurons is likely to depend on laminar location. It will be important for future studies to examine how interneuron subtypes in different cortical layers contribute to sensory processing. The use and care of animals complied with the guidelines of the Animal Advisory Committee at the Shanghai Institutes for Biological Sciences, and all experiments were approved by the Animal Care and Use Committee at the Institute of Neuroscience, Chinese Academy of Sciences. Virus injections and head-plate implant Adult PV-Cre (The Jackson Laboratory, stock no. 008069) or SOM-Cre (stock no. 013044) mice (both sexes, 2–6 months) were anaesthetized with ketamine (200 mg kg −1 ) and xylazine (10 mg kg −1 ) or a mixture of midazolam (5 mg kg −1 ), fentanyl (0.05 mg kg −1 ) and medetomidin (0.5 mg kg −1 ). A small craniotomy (<500 μm diameters) was made over V1 (3.2 mm posterior from bregma, 2.2 mm lateral to the midline). The virus (AAV-FLEX-ArchT-GFP) was filled into a glass pipette (20–40 μm tip diameter) and 1 μl of virus (containing>1 × 10 9 viral particles) was injected at a depth of 500–750 μm below the pia at a rate of 0.03–0.1 μl min −1 using a syringe pump (Harvard Apparatus). After the completion of virus injection, the pipette was held in place for at least 10 min before retraction. For recordings in awake mice, a stainless-steel head plate was cemented to the skull with dental acrylic after the virus injection. Antiphlogistic drug (ceftriaxone sodium, 2 mg kg −1 , intramuscular injection) was administered after the surgery. The skull over the virus injection site was covered by silicon elastomer (Kwik-Cast, WPI). Immunohistochemistry The mice were deeply anaesthetized with ketamine and were transcardially perfused with saline followed by ∼ 20 ml of a fixative containing 4% paraformaldehyde. The brain was removed from the skull, postfixed in 4% paraformaldehyde overnight (4 °C) and then transferred to 30% sucrose in PBS solution. Brains were embedded in OCT compound (Sakura, 4583) and sectioned into 40-μm coronal slices using a cryostat (Microm). Slices were incubated in the blocking buffer (5% BSA, 0.5% Triton X-100 in PBS) for 2 h at room temperature and then in primary antibodies diluted in blocking buffer overnight at 4 °C. For double-labelling immunofluorescence, we used the primary antibody for green fluorescent protein (GFP) (rabbit anti-GFP, 1:1,000, Invitrogen, A11122), with antibody for PV (guinea pig anti-PV, 1:500, SYSY, 195 004) or for somatostatin (goat anti-somatostatin, 1:200, Santa Cruz Biotech, sc-7819). Slices were then washed with PBS three times every 10 min and incubated in blocking buffer diluted with specific secondary antibodies for PV (donkey anti-guinea pig-Cy3, 1:500, Jacksonimmuno, 706-166-148) or somatostatin (donkey anti-goat Alexa Fluor 546, 1:500, Invitrogen, A11056) and GFP (donkey anti-rabbit Alexa Fluor 488, 1:1,000, Invitrogen, A21206) for 2 h at room temperature. Slices were washed three times with PBS and mounted on slides and coverslipped with Vectashield (Vector, H-1000) or Mowiol 4–88 (Calbiochem, 475904). Images of immunofluorescent slices were taken with a fluorescence confocal microscope (Zeiss, Nikon, or Olympus). To observe the laminar pattern of Arch-GFP expression, we used Hoechst 33342 to identify the cellular nuclei. In vivo recordings Recordings were made at least 3 weeks after the virus injection. For PV suppression, we performed a total of 25 and 32 experiments from anaesthetized and awake mice, respectively. For SOM suppression, we performed a total of 12 and 23 experiments from anaesthetized and awake mice, respectively. For PV or SOM suppression experiment, we collected enough data to guarantee the validity of the statistical test. For anaesthetized recordings, mice were sedated with an intraperitoneal injection of chlorprothixene (5 mg kg −1 ) and then anaesthetized with urethane (1.0–1.2 g kg −1 ). The animals were restrained in a stereotaxic apparatus and their body temperature was maintained at ∼ 37.5 °C by a heating pad. Silicon oil was applied to the eyes, to prevent from drying. A craniotomy ( ∼ 1 mm diameter) was performed over V1 near the virus injection site and dura was removed. For awake recordings, the head plate of the mouse was fixed to a holder attached to the stereotaxic apparatus and the mouse’s body was restricted in an acrylic tube. Following anaesthesia with isoflurane ( ∼ 1%), a craniotomy was performed. The animal was allowed to recover from the anaesthesia for at least 1 h. The exposed cortex of awake mice was covered by 2.5% agar to improve stability (and the agar reduced the actual laser power by ∼ 20%). A 16-channel silicon probe (A1 × 16-3 mm-50-177, 50 μm between sites, Neuronexus Technologies) was inserted perpendicularly into V1. The probe was inserted at least 200 μm away from the virus injection site in which successful expression of Arch-GFP was confirmed by the fluorescent signal under a microscope. For anaesthetized experiments, the reference electrode was placed in the frontal cortex and the ground electrode was placed under the skull above the frontal cortex. For awake experiments, both reference and ground electrodes were wrapped around a screw in the frontal cortex. The responses were amplified and filtered using a Cerebus 32-channel system (Blackrock Microsystems). LFP signals were sampled at 2 kHz per channel with a wide-band front-end filter (0.3–500 Hz). Spiking signals were sampled at 30 kHz. To detect spike waveforms, we band-pass filtered the signals at 250–7,500 Hz and set a threshold at 4 s.d. of the background noise. Visual stimulation Visual stimuli were presented with a 7" or 17" LCD monitor (refresh rate 60 Hz; mean luminance 97.3 or 40 cd m −2 ) placed 35 or 100 mm from the contralateral eye. All stimuli were updated every two frames, resulting in an effective frame rate of 30 Hz. Movie clips were selected from the van Hateren natural movie database [51] . Each trial of movie presentation consisted of a 6-s or 3-s movie (180 or 90 frames, 64 × 64 pixels, RMS contrast of 0.29) followed by 5-s blank grey screen (150 frames). During movie stimulation, control trials (20–40 repeats) were interleaved with photo stimulation trials (20–40 repeats). In the experiments using awake mice, following the movie stimulation we presented 20 trials of 6-s or 3-s blank grey screen (control trials interleaved with photo stimulation trials). The RF was measured using sparse noise stimuli, in which a white square (11° × 11°–15° × 15°) was flashed for 33.3 ms on a black background at each of the 7 × 7 positions in a pseudorandom sequence for 100 repeats. The sizes of the movie stimuli were 53° × 53°–73° × 73°, covering the RFs of all units in the same recording. Two types of stimuli were used to measure the visual responses used for CSD analysis. In some experiments, we displayed 600 repeats of flash stimuli (102° × 102°, 100% contrast) for 500 ms with an interval of 500 ms. In other experiments, we presented sparse noise stimuli (7 × 7, 100 repeats) and used the responses to light squares (11° × 11°–15° × 15°) flashed within the RF of the neurons to compute CSD. Optogenetic photo stimulation Photo suppression by Arch activation was achieved using a green laser (532 nm; Shanghai Laser & Optics Century Co.) connected to an output optic fibre (50 μm core diameter; 0.13 NA). The laser was switched on and off by a Master-9 pulse stimulator (A.M.P.I.). The light passed through a collimator and was focused on the cortical surface around the probe insertion site. For each experiment, light intensity was adjusted to a level at which photo perturbation of spontaneous firing rate was detectable (10% ∼ 40% increase in the multi-unit activity). The increase in spontaneous response was not significantly different between broad-spiking cells in PV and SOM suppression experiments ( Supplementary Fig. 1i ). For the PV suppression experiment, light intensity was also carefully adjusted not to be too large to cause epileptiform activity in the LFP ( Supplementary Fig. 2 ). Light intensities were in the range of 1–17 mW (with most experiments <5 mW). For trials of photo stimulation, laser was turned on 0.5 s before the onset of visual stimuli and turned off 0.5 s after the termination of stimuli. To ensure that photo stimulation itself (without Arch) did not influence V1 responses, we also performed control experiments on PV-Cre mice in which the virus was not injected. Data analysis Spikes recorded in each contact of the multi-site probe were independently sorted with the Offline Sorter (Plexon Inc.) using cluster analysis of principal component amplitudes ( Supplementary Fig. 13 ). Spike clusters were considered to be single units if few spikes (<0.3%) had an interspike interval <1 ms and P <0.05 for multivariate analysis of variance tests on clusters. To determine whether the same spikes appear in multiple channels, we computed CCs (binned at 1 ms) between all pair-wise combinations of units recorded in the same electrode. Those pairs with a CC>0.1 were considered to contain duplicate units and the unit with the lower firing rate in the pair was discarded [36] . Based on the spike waveforms, units were classified as broad spiking or narrow spiking, corresponding to putative excitatory or putative inhibitory neurons [34] , respectively. For each unit, all spikes were aligned by their troughs and averaged. To facilitate the computation of waveform parameters, the average waveform of each unit was interpolated [52] . Average waveforms of all units were then aligned by their troughs and normalized by trough depth. Two parameters were computed: the slope of the waveform 0.4–0.6 ms after the initial trough [34] and the width of the peak at half-maximum of the peak amplitude [52] . Two clusters were identified using fuzzy c-means clustering. For the two populations of broad-spiking cells sampled from PV and SOM suppression experiments, neither the waveform slopes nor the waveform widths were significantly different ( Supplementary Fig. 1e,f ). To compute the spontaneous responses for the experiments of anaesthetized mice, we used the responses occurring in a 500-ms window preceding each trial of the movie stimulus. In the experiments of awake mice, following the movie stimulation we presented 20 trials of 6-s or 3-s blank grey screen (control trials interleaved with photo stimulation trials) and we used the responses to these blank screens as spontaneous. For the responses to sparse noise, the spikes were binned at stimulus frame rate and RF maps were obtained by cross-correlating the spike responses with the sparse noise stimuli [53] . For the movie-evoked responses, the spike trains were binned at the stimulus frame rate (corresponding to 33.3 ms) or several other bin sizes (20, 100, 200 and 300 ms). To quantify the reliability of movie responses, we computed the average between-trial Pearson CC [36] . To determine whether a neuron was visually driven, we separated the movie into two segments (for example, separated a 6-s movie into two 3-s segments) and computed the average between-trial CCs (responses binned at the stimulus frame rate) within segment and between segments [36] . Only those cells that had significantly higher within-segment CCs ( P <0.01, Wilcoxon signed-rank test) and firing rate>1 spike per second were included in the analyses. For SOM suppression experiments, the firing rates of three broad-spiking cells were significantly decreased after photo stimulation ( P <0.01, Wilcoxon signed-rank test). We excluded the three cells from the analysis, because SOM-expressing interneurons are broad spiking [54] and these three cells could be SOM-expressing interneurons that were directly suppressed by photo stimulation of Arch. Based on the above criteria, the number of broad-spiking cells included in the analysis were 98 (from 23 experiments), 28 (from 18 experiments), 51 (from 11 experiments) and 25 (from 14 experiments) for PV suppression in anaesthetized mice, PV suppression in awake mice, SOM suppression in anaesthetized mice and SOM suppression in awake mice, respectively. The CC change (ΔCC) induced by photo stimulation was computed as CC measured with photo stimulation minus that without photo stimulation. The ΔRate was computed as R light −R control , and the percent change in firing rate as ( R light −R control )/ R control , where R control and R light represent firing rates during control trials and photo stimulation trials, respectively. For the movie-evoked PSTH (binned at the stimulus frame rate) measured in control trials, we set a threshold at 25% of the highest amplitude of the PSTH and defined events (non-events) as those time bins above (below) the threshold [38] . SNR was defined as the ratio between mean response of events and s.d. of event responses over trials [29] . The change in SNR (ΔSNR) was computed as SNR light −SNR control , where SNR control and SNR light represent SNRs during control trials and photo stimulation trials, respectively. FF of the events was computed as the time average of the ratio between spike count variance and mean spike count. To examine whether the change in CC may result from the increase in firing rates, we performed a spike rate equalization analysis [36] . For each pair of trials with and without photo stimulation, the firing rates were equalized by randomly adding spikes for the spike train with lower firing rate. The between-trial CCs were computed for the responses after spike rate equalization. For each neuron, the spike rate equalization was repeated 3,000 times and these CCs were averaged. Response sparseness was computed as , where n is the total number of time bins of the PSTH (binned at the stimulus frame rate) and r i is the firing rate at the i -th bin [9] , [39] . Sparseness is a nonparametric measure of neuronal selectivity and makes no assumption about the form of firing rate distribution, the tuning properties of the neuron and the number of stimuli in the set [55] . The change in sparseness was computed as sparseness measured with photo stimulation minus that without photo stimulation. To examine the relationship between the firing rates with and without photo stimulation, we binned the responses at 300 ms and used the robustfit function in Matlab statistics toolbox to perform robust linear regression. To compare the effects of PV and SOM suppression on CC, we used the aoctool function in Matlab to perform analysis of covariance. To determine the relationships among changes in CC, event firing rate and SNR for PV suppression, or the relationships among changes in sparseness, firing rate and CC, we computed partial correlations using the partialcorr function in Matlab. To determine the location of layer 4, we measured the LFP responses to flash stimuli for all 16 recording sites. LFP traces were band-pass filtered between 1 and 300 Hz [34] , and CSD profiles were computed from the filtered LFP [56] , [57] . We first converted the 16 recording sites to 18 sites by duplicating the LFP trace of the most superficial site and the deepest site [58] , [59] . We next smoothed the LFP traces for 16 of the 18 sites (from the 2nd to the 17th site) [58] : where φ is LFP, z is the coordinate of the recording sites, Δ z is the distance between adjacent recording sites (50 μm) and n Δ z is the differentiation grid ( n =1). We then used the 18 LFP traces to compute the second spatial derivative of LFP [56] , [57] : where φ is LFP, z is the coordinate of the recording sites, Δ z is the distance between adjacent recording sites and n Δ z is the differentiation grid ( n =2). This generated CSD profiles of 14 channels. Layer 4 (the granular layer) was determined as the recording sites at the initial current sink and assumed to be ∼ 150 μm wide, and the supragranular and infragraular layers were those above and below layer 4. As the electrode was lowered into the cortex, the location of current sink moved along the electrode ( Supplementary Fig. 8a ), demonstrating that the initial current sink can be used to locate layer 4. To confirm the width of layer 4, we performed Nissl staining for the coronal sections of brain containing V1. For PV-Cre mouse, the average thickness of layer 2/3, layer 4 and layer 5/6 of V1 was 212±19, 148±11 and 417±28 μm, respectively (s.d., n =4 brains, 25 locations). For SOM-Cre mouse, the average thickness of layer 2/3, layer 4 and layer 5/6 of V1 was 207±22, 150±28 and 401±39 μm, respectively (s.d., n =4 brains, 20 locations). For the laminar analysis, only those recordings whose laminar locations could be determined from the CSD analysis were used. For the broad-spiking cells included in the analysis, we could determine the laminar locations for 16 experiments in anaesthetized mice and 16 experiments in awake mice for PV suppression, and 11 experiments in anaesthetized mice and 12 experiments in awake mice for SOM suppression. Neural discrimination was quantified based on classification analysis [40] , [41] . The 6- or 3-s movie was divided into multiple segments (200 ms per segment). For each segment, we used the averaged response across trials as the response template. The given trial used for discrimination was not included to compute the template [40] . A single-trial response to a given movie segment was compared with the template in each segment on the basis of Euclidean distance: where x i denotes a single-trial response and represents a template. The single-trial response was classified to the segment that yielded the minimum distance. Discrimination performance was computed as the proportion of correct classifications. How to cite this article: Zhu, Y. et al , Control of response reliability by parvalbumin-expressing interneurons in visual cortex. Nat. Commun , 6:6802 doi: 10.1038/ncomms7802 (2015).